Radial-arrayed rotary electrification for high performance triboelectric generator Harvesting mechanical energy is an important route in obtaining cost-effective, clean and sustainable electric energy. Here we report a two-dimensional planar-structured triboelectric generator on the basis of contact electrification. The radial arrays of micro-sized sectors on the contact surfaces enable a high output power of 1.5 W (area power density of 19 mW cm −2 ) at an efficiency of 24%. The triboelectric generator can effectively harness various ambient motions, including light wind, tap water flow and normal body movement. Through a power management circuit, a triboelectric-generator-based power-supplying system can provide a constant direct-current source for sustainably driving and charging commercial electronics, immediately demonstrating the feasibility of the triboelectric generator as a practical power source. Given exceptional power density, extremely low cost and unique applicability resulting from distinctive mechanism and structure, the triboelectric generator can be applied not only to self-powered electronics but also possibly to power generation at a large scale. The quality of life and sustainable development of modern society are largely defined by the available amount of electric power. Everything that hallmarks the high-tech era, from advanced illumination through smart appliances to portable and even wearable electronics, depends on electricity, which has become indispensable in people’s daily life. Although electricity-generating technologies have been developed for two hundred years, people have never ceased to explore new methods through different mechanisms including photoelectric effect [1] , [2] , [3] , piezoelectric effect [4] , [5] , [6] , thermoelectric effect [7] , [8] , [9] , electrochemical reaction [10] , [11] , [12] and electrostatic induction [13] , [14] , [15] , among others, in order to address the rapidly rising demand on electric power. Among them, harvesting mechanical energy is attracting increasing attentions due to the extensive availability of the target resource [16] , [17] , [18] , [19] , [20] , [21] , [22] , [23] , [24] , [25] . Recently we have introduced a new concept on the basis of triboelectrification for harvesting energy from various ambient mechanical motions [26] , [27] , [28] . However, a breakthrough is desperately needed to boost the output power so that it can be used as an effective power source for practical applications. Therefore, it is critical to explore advanced designs and approaches. Besides, other practical issues such as high output impedance, mechanical fragility, fluctuation in output power and alternating current (AC) output also need to be properly addressed before the triboelectrification-based generator becomes a truly practical new energy technology. In this communication we report a triboelectric generator (TEG) for producing energy from rotary surfaces with unprecedented performance. Enabled by a design of two radial-arrayed fine electrodes that are complementary on the same plane, the planar-structured TEG generates periodically changing triboelectric potential that induces ACs between electrodes. Operating at a rotation rate of 3,000 r min −1 , a TEG having a diameter of 10 cm can produce an open-circuit voltage ( V oc ) of ~850 V and a short-circuit current ( I sc ) of ~3 mA at a frequency of 3 KHz. Under the matched load of 0.8 MΩ, an average output power of 1.5 W (an area power density of 19 mW cm −2 ) can be delivered to an external load at an efficiency of 24%, representing a gigantic leap in terms of output power by orders of magnitude compared with previous reports [29] , [30] . The TEG is demonstrated as an effective measure in harvesting a variety of ambient mechanical motions, such as light wind, water flow and body movement. More importantly, a complete power-supplying system is built through integrating a power management circuit with the TEG, which can provide a continuous direct-current (DC) source at a constant voltage for sustainably driving as well as charging various commercial electronics and thus immediately demonstrate the feasibility of the TEG as a practical technology. Given other compelling features of the TEG including small volume, light weight, low cost and proven scalability, it is not only suited to harvest mechanical energy for self-powered electronics, but also it can be potentially applied to large-scale energy generation. Device structure A TEG has a multilayered structure, which consists of mainly two parts, that is, a rotator and a stator, as sketched in Fig. 1a . The rotator is a collection of radially-arrayed sectors separated by equal-degree intervals in between. With each sector unit having a central angle of 3°, the rotator has a total of 60 units. For the stator, it is divided into three components. A layer of fluorinated ethylene propylene (FEP) as an electrification material, a layer of electrodes and an underlying substrate are laminated along the vertical direction. The electrode layer is composed of two complementary-patterned electrode networks that are disconnected by fine trenches in between ( Fig. 1b,c ). Having the same pattern as that of the rotator, each network is formed by a radial array of sectors that are mutually connected at one end. The electrode layer is fully imbedded and stationary. This rational design not only leads to structural simplicity but also accounts for excellent robustness, making the TEG practically reliable and durable. As exhibited in Fig. 1d,e , both the rotator and the stator have two-dimensional planar structures, respectively, resulting in a small volume of the TEG. Detailed fabrication process is discussed in Methods. 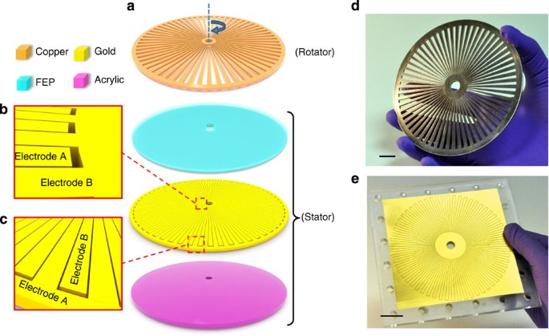Figure 1: Structural design of the triboelectric generator. (a) Schematic illustrations of the triboelectric generator, which has two parts, that is, a rotator and a stator. The zoomed-in illustrations at the inner end (b) and the outer end (c) reveal that the two electrodes have complementary patterns, which are separated by fine trenches in between. It is noted that these drawings do not scale. (d) Photograph of a rotator (scale bar, 1 cm). (e) Photograph of a stator, in which the through-holes along edges are for mounting purpose (scale bar, 2 cm). Figure 1: Structural design of the triboelectric generator. ( a ) Schematic illustrations of the triboelectric generator, which has two parts, that is, a rotator and a stator. The zoomed-in illustrations at the inner end ( b ) and the outer end ( c ) reveal that the two electrodes have complementary patterns, which are separated by fine trenches in between. It is noted that these drawings do not scale. ( d ) Photograph of a rotator (scale bar, 1 cm). ( e ) Photograph of a stator, in which the through-holes along edges are for mounting purpose (scale bar, 2 cm). Full size image Electricity generation process The operation of the TEG relies on relative rotation between the rotator and the stator, in which a unique coupling between triboelectrification and electrostatic induction gives rise to alternating flow of electrons between electrodes. The electricity-generating process is elaborated through a basic unit in Fig. 2 . We define the initial state ( Fig. 2a ) and the final state ( Fig. 2c ) as the states when the rotator is aligned with electrode A and electrode B, respectively. The intermediate state ( Fig. 2b ) represents the transitional process in which the rotator spins from the initial position to the final position. Since the rotator and the stator are in direct contact, triboelectrification creates charge transfer on contacting surfaces, with negative charges generated on the FEP and positive ones on the metal [29] , [31] , as illustrated in the cross-sectional view defined by an arbitrary intersection in Fig. 2 . Due to the law of charge conservation, the density of positive charges on the rotator is twice as much as that of negative ones on the stator because of unequal contact surface area of the two objects. 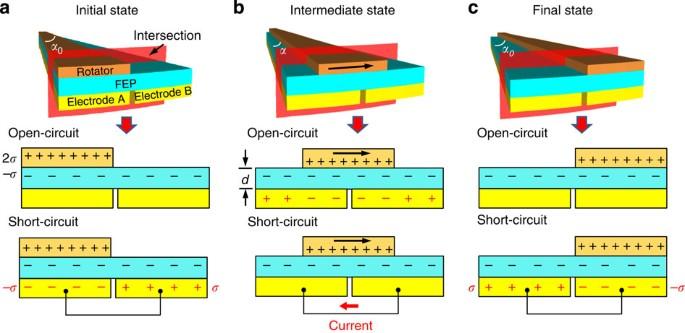Figure 2: Schematics of operating principle of the triboelectric generator. (a) Initial state in which the rotator is in alignment with electrode A. The three sections from top to bottom illustrate the three-dimensional schematic, charge distribution in open-circuit condition, and charge distribution in short-circuit condition, respectively. (b) Intermediate state in which the rotator is spinning away from the initial position at an angle ofα. (c) Final state in which the rotator is in alignment with electrode B. The rotator has rotatedα0away from the initial position. Figure 2: Schematics of operating principle of the triboelectric generator. ( a ) Initial state in which the rotator is in alignment with electrode A. The three sections from top to bottom illustrate the three-dimensional schematic, charge distribution in open-circuit condition, and charge distribution in short-circuit condition, respectively. ( b ) Intermediate state in which the rotator is spinning away from the initial position at an angle of α . ( c ) Final state in which the rotator is in alignment with electrode B. The rotator has rotated α 0 away from the initial position. Full size image In open-circuit condition, electrons cannot transfer between electrodes. The open-circuit voltage is then defined as the electric potential difference between the two electrodes, that is, V oc = U A − U B . The initial state corresponds to the maximum potential on electrode A and the minimum potential on electrode B, which results in the maximum V oc . Such a voltage then diminishes as the rotator starts to spin. Once the rotator passes the middle position, V oc with the opposite polarity starts to build up until the rotator reaches the final state. Further rotation beyond the final state induces the V oc to change in a reversed way because of the periodic structure. The continuous variation of the V oc is visualized via COMSOL in Supplementary Movie 1 . On the basis of the assumption that the thickness of the dielectric layer is far smaller than the width dimension in Fig. 2 , an analytical model can be established, in which any overlapped region between the rotator and the electrodes can be treated as a parallel-plate capacitor without consideration of edge effect [15] , [32] . Then the V oc can be analytically expressed by the following equations using Gauss Theorem. The detailed model is presented in Supplementary Fig. 1 and Supplementary Note 1 . where d is the thickness of the FEP layer, σ is the triboelectric charge density on top of the FEP layer, ε 0 is the dielectric constant of vaccum, ε r is the relative dielectric constant of FEP, α is the angle at which the rotator rotates away from the initial state, and α 0 is the central angle of a single rotator unit. The equation (2) can only be used to illustrate the changing trend of the V oc (see Supplementary Note 1 ). The theoretical peak-to-peak value of the V oc needs to be calculated by subtracting equation (3) from equation (1): By substituting the known parameters into equation (4) ( d =25 μm, σ =~200 μC m −2 , ε r =2.1) [29] , the V oc (peak-to-peak) is theoretically estimated to be ~1,000 V. If the two electrodes are connected as shown by the bottom row in Fig. 2 , free charges can redistribute between electrodes due to electrostatic induction. At the initial state, induced charges accumulate on electrode A and electrode B with charge density of − σ and σ , respectively. As the rotation starts, free electrons keep flowing from electrode A to electrode B until the rotator reaches the final state where the charge density on both electrodes is reversed in polarity compared with the initial state. As a result, the amount of charges in this transport process can be expressed by the following equation where r 2 and r 1 are the outer radius and inner radius of the TEG, respectively. Again, further rotation beyond the final state results in a current in the opposite direction (see Supplementary Fig. 2 and Supplementary Note 2 for detailed derivations). Therefore, AC is generated as a result of the periodically changing electric field, which has a frequency calculated as where ν is the rotation rate (r sec −1 ). Electric measurement To control the rotation rate for quantitative measurement, a programmable rotary motor was connected to the rotator that was in coaxial alignment with the stator. At a rotating rate of 500 r min −1 , short-circuit current ( I sc ) has a continuous AC output at an average amplitude of 0.5 mA ( Fig. 3a ). The constant frequency of 500 Hz is consistent with the result calculated from equation (6). For open-circuit voltage ( V oc ), it oscillates at the same frequency as that of I sc with a peak-to-peak value of 870 V ( Fig. 3b ), which corresponds well to the theoretical value obtained from equation (4) though the slight deviation is likely attributed to the fact that the actual contact area is less than the apparent device area because of surface roughness. In short-circuit condition, the amount of electrons in a single electron-transport process reaches 0.32 μC ( Fig. 3c ), which corresponds to an effective DC current ( I dc =Δ Q/ Δ t ) of 0.32 mA. It is noticed that the duration of a current peak is determined by the ratio between the central angle of a sector and the rotation rate ( Fig. 3a ). Once an external load is applied, the amplitude of the output current drops as the load resistance increases, as shown in Fig. 3d . The average output power is equivalent to the Joule heating of the load resistor, which can be calculated as , where I effective is the effective current defined as the root mean square value of the current amplitude, and R is the load resistance. At the matched load of 4.9 MΩ, the average output power reaches 0.23 W at a rotation rate of 500 r min −1 ( Fig. 3d ). 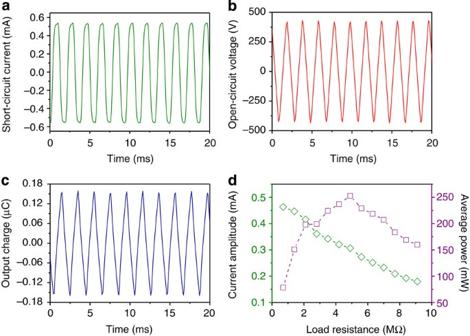Figure 3: Results of electric measurements. (a) Short-circuit current (Isc) at a rotation rate of 500 r min−1. (b) Open-circuit voltage (Voc) at a rotation rate of 500 r min−1. (c) Output charge at a rotation rate of 500 r min−1. (d) Load matching test at a rotation rate of 500 r min−1. Maximum average output power is obtained at the matched load of 4.9 MΩ. Figure 3: Results of electric measurements. ( a ) Short-circuit current ( I sc ) at a rotation rate of 500 r min −1 . ( b ) Open-circuit voltage ( V oc ) at a rotation rate of 500 r min −1 . ( c ) Output charge at a rotation rate of 500 r min −1 . ( d ) Load matching test at a rotation rate of 500 r min −1 . Maximum average output power is obtained at the matched load of 4.9 MΩ. Full size image Tuning output power Rotation rate is a major factor that determines electric output of the TEG. A linear relationship can be derived from Fig. 4a between the amplitude of I sc and the rotation rate since higher rate linearly shortens the duration of a current peak and thus boosts the current amplitude. In comparison, the amplitude of V oc remains stable regardless of the rotation rate ( Fig. 4a ) because it is only dependent on the position of the rotator, as indicated in equation (2). It is found that the matched load is also a variable value, exhibiting a reversely proportional relationship with the rotation rate, as diagrammed in Fig. 4b . Consequently, linearly rising output power can be obtained at higher rotation rate ( Fig. 4b ). Given the linear behaviour of the TEG, it delivers an optimum average output power of ~1.5 W at the matched load of ~0.8 MΩ when operating at a rotation rate of 3,000 r min −1 , which corresponds to an average output power density of 19 mW cm −2 . For the first time, the output power from triboelectrification-based generators is boosted to a level where it is sufficiently powerful to drive daily used electronics, immediately resolving the most critical concern for the concept of power generation via triboelectrification. 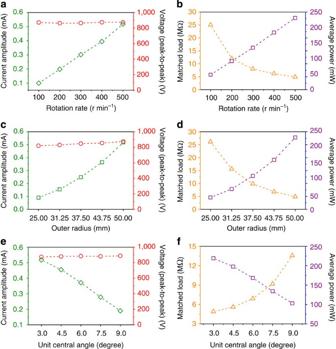Figure 4: Factors that influence the electric output of the triboelectric generator. (a) Amplitude ofIscand peak-to-peak value ofVocwith increasing rotation rate. (b) Matched load resistance and average output power with increasing rotation rate. (c) Amplitude ofIscand peak-to-peak value ofVocwith increasing outer radius of the triboelectric generator (500 r min−1). (d) Matched load resistance and average output power with increasing outer radius of the triboelectric generator (500 r min−1). (e) Amplitude ofIscand peak-to-peak value ofVocwith increasing central angle of a unit sector (500 r min−1). (f) Matched load resistance and average output power with increasing central angle of a unit sector (500 r min−1). Figure 4: Factors that influence the electric output of the triboelectric generator. ( a ) Amplitude of I sc and peak-to-peak value of V oc with increasing rotation rate. ( b ) Matched load resistance and average output power with increasing rotation rate. ( c ) Amplitude of I sc and peak-to-peak value of V oc with increasing outer radius of the triboelectric generator (500 r min −1 ). ( d ) Matched load resistance and average output power with increasing outer radius of the triboelectric generator (500 r min −1 ). ( e ) Amplitude of I sc and peak-to-peak value of V oc with increasing central angle of a unit sector (500 r min −1 ). ( f ) Matched load resistance and average output power with increasing central angle of a unit sector (500 r min −1 ). Full size image Design parameters, especially the size and the unit central angle, can also largely influence the output power of the TEG. Figure 4c shows an approximately quadratic dependence of the I sc and independence of the V oc on the radius of the TEG, which are consistent with the results in equations (4) and (5), respectively. With the matched load decreasing with the radius, the average output power exhibits a roughly quadratic relationship with the radius ( Fig. 4d ). In other words, the output power linearly scales with the area of the TEG since the triboelectrification is a surface charging effect that is area-dependent. Compared with the device size, the unit central angle reversely affects the output power. As revealed in Fig. 4e , the I sc linearly drops as the central angle increases, while the V oc still remains stable. Again, the measured results fit well with the theoretical model. Consequently, the average output power decreases in almost a linear way if devices with larger central angle are used ( Fig. 4f ). Therefore, fine feature size of the unit sector plays a key role in achieving high output power. Efficiency and reliability The efficiency of the TEG is defined as the ratio of the input mechanical power from the motor to the electric power that is delivered to the load. When driving the TEG at a rotation rate of 3,000 r min −1 , the motor exhibits a load factor of approximately 20%, corresponding to an actual torque of 0.02 N m delivered to the TEG. Then we can derive the power input from the motor to be 6.28 W by using the above values. Given the electric output power of 1.5 W at the same rotation rate, the efficiency is calculated to be ~24%. The reliability of the TEG, especially the resistance against mechanical wear, is important in evaluating its performance. Here, adhesive wear that occurs when two nominally flat solid bodies are in sliding contact applies to the TEG [33] . Therefore, the adhesion of the deposited metal on the rotator largely determines the wear resistance. Special treatment was taken in fabricating the TEG, including adding an adhesion layer and surface plasma treatment before metal deposition [34] , [35] . As a result, the TEG shows excellent stability and durability. After continuously producing more than 10 million cycles of AC, the output current does not even exhibit any measurable decay or degradation ( Supplementary Fig. 3 ), which firmly proves the reliability of the TEG as a feasible approach for practical applications. Power source for electronics To demonstrate the capability of the TEG as a power source, it was directly connected to regular light bulbs without using a storage or power regulation unit. The rotation rate was set at 1,000 r min −1 . A total of 20 spot lights were simultaneously lighted up ( Fig. 5a , Supplementary Movie 2 ), providing sufficient illumination even for reading printed text in complete darkness ( Fig. 5b , Supplementary Movie 3 ). Moreover, other types of light bulbs that could be driven by the TEG included a white globe light ( Fig. 5c , Supplementary Movie 4 ) and 10 multicolor decoration candelabra lights ( Fig. 5d , Supplementary Movie 5 ). 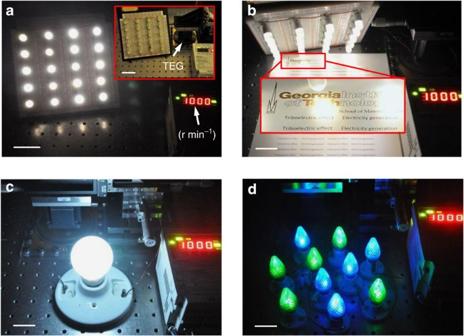Figure 5: Demonstrations of the triboelectric generator as a practical power source. (a) Photograph of 20 spot lights that are directly powered by the triboelectric generator in complete darkness (rotation rate: 1,000 r min−1; scale bar, 5 cm). Inset: demonstration setup (scale bar, 5 cm). (b) Photograph of printed text on a paper illuminated by the 20 spot lights in complete darkness with the triboelectric generator as a direct power source (rotation rate: 1,000 r min−1; scale bar, 3 cm). The font size is 12 points. (c) Photograph of a G16 globe light that is directly powered by the triboelectric generator in complete darkness (rotation rate: 1,000 r min−1; scale bar, 3 cm). (d) Photograph of 10 multicolor decoration candelabra lights that are directly powered by the triboelectric generator in complete darkness (rotation rate: 1,000 r min−1; scale bar, 3 cm). Figure 5: Demonstrations of the triboelectric generator as a practical power source. ( a ) Photograph of 20 spot lights that are directly powered by the triboelectric generator in complete darkness (rotation rate: 1,000 r min −1 ; scale bar, 5 cm). Inset: demonstration setup (scale bar, 5 cm). ( b ) Photograph of printed text on a paper illuminated by the 20 spot lights in complete darkness with the triboelectric generator as a direct power source (rotation rate: 1,000 r min −1 ; scale bar, 3 cm). The font size is 12 points. ( c ) Photograph of a G16 globe light that is directly powered by the triboelectric generator in complete darkness (rotation rate: 1,000 r min −1 ; scale bar, 3 cm). ( d ) Photograph of 10 multicolor decoration candelabra lights that are directly powered by the triboelectric generator in complete darkness (rotation rate: 1,000 r min −1 ; scale bar, 3 cm). Full size image It is noticed that the TEG has high voltage but relatively low current, resulting in large output impedance and thus affecting its applicability as a power source. Besides, fluctuation in output power and the AC output current are also concerns in practical applications. These issues can be fully addressed by integrating the TEG with a power management circuit to form a complete power-supplying system. Consisting of a transformer, a rectifier, a voltage regulator and capacitors, the power management circuit as diagrammed in Fig. 6a can deliver a DC output at a constant voltage of 5 V in less than 0.5 s after the TEG starts to operate ( Fig. 6b ). The transformer shown in Fig. 6a is able to tremendously boost the output current at the expense of the output voltage ( Supplementary Fig. 4 ), which substantially reduces the output impedance of the TEG. The power-supplying system is suited to a variety of purposes. On one hand, it could provide a continuous uniform DC power to drive various commercial electronics. As demonstrated in Fig. 6c and Supplementary Movie 6 , 10 LED bulbs (0.75 mW each) connected parallel to output terminals of the circuit were continuously powered with full brightness. Moreover, once the output voltage reaches 5 V, the power-supplying system could sustain wireless transmissions for five times ( Fig. 6d , Supplementary Fig. 5 , Supplementary Movie 7 ) as well as continuous operation of a multifunction digital clock for 60 s ( Fig. 6e , Supplementary Fig. 6 , Supplementary Movie 8 ). On the other hand, the system is also able to serve as a charging source for batteries. Since 5 V is the standard charging voltage for most of the commercial portable electronics, a cellphone automatically turned on once the voltage output shot to 5 V due to the operation of the TEG, as visualized in Fig. 6f , Supplementary Fig. 7 and Supplementary Movie 9 . 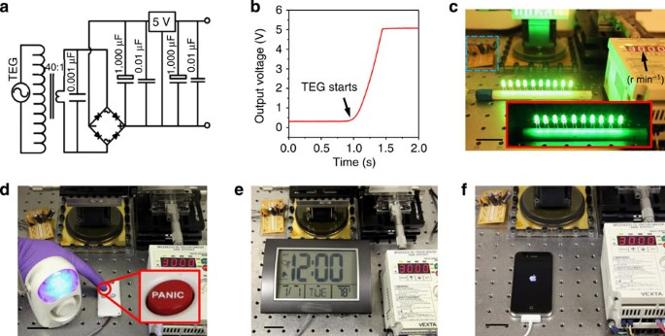Figure 6: Demonstrations of the integrated power-supplying system for driving and charging electronics. (a) Circuit diagram of the complete power-supplying system that consists of a triboelectric generator and a power management circuit. (b) Output voltage of the system reaches a constant value of 5 V in less than 0.5 s as the triboelectric generator starts to rotate at 3,000 r min−1. (c) Photograph of 10 LEDs (0.75 mW each) in parallel that are powered to full brightness by the power-supplying system with ambient background lighting (rotation rate: 3,000 r min−1; scale bar, 3 cm). The dashed blue box indicates the power management circuit. Inset: photograph of the lighted LEDs in complete darkness. (d) Photograph of an alarm triggered by a wireless emitter that relies on the power-supplying system (scale bar, 3 cm). Inset: photograph of the ‘panic’ button that sets off the alarm. (e) Photograph of a multifunction digital clock driven by the power-supplying system (scale bar, 3 cm). (f) Photograph of a cellphone that is being charged by the power-supplying system (scale bar, 3 cm). As soon as the output voltage of the system reaches 5 V, the cellphone turns on automatically. Figure 6: Demonstrations of the integrated power-supplying system for driving and charging electronics. ( a ) Circuit diagram of the complete power-supplying system that consists of a triboelectric generator and a power management circuit. ( b ) Output voltage of the system reaches a constant value of 5 V in less than 0.5 s as the triboelectric generator starts to rotate at 3,000 r min −1 . ( c ) Photograph of 10 LEDs (0.75 mW each) in parallel that are powered to full brightness by the power-supplying system with ambient background lighting (rotation rate: 3,000 r min −1 ; scale bar, 3 cm). The dashed blue box indicates the power management circuit. Inset: photograph of the lighted LEDs in complete darkness. ( d ) Photograph of an alarm triggered by a wireless emitter that relies on the power-supplying system (scale bar, 3 cm). Inset: photograph of the ‘panic’ button that sets off the alarm. ( e ) Photograph of a multifunction digital clock driven by the power-supplying system (scale bar, 3 cm). ( f ) Photograph of a cellphone that is being charged by the power-supplying system (scale bar, 3 cm). As soon as the output voltage of the system reaches 5 V, the cellphone turns on automatically. Full size image Operation in ambient environment In addition to being driven by an electric motor for quantitative measurement, the TEG was further tested in normal environment where a series of ambient mechanical energy was harvested. First, energy harvesting from light air flow (wind) was demonstrated ( Fig. 7a ). Artificial breeze was generated at a speed of 6 m s −1 by an air mover. The wind perpendicularly blew on a miniaturized three-vane wind turbine (inset in Fig. 7a ). Driven by the turbine through a transmission shaft, the rotator of the TEG spun smoothly, directly providing a power source for lighting up an array of spot lights ( Supplementary Movie 10 ). Such a wind speed falls into class 4 defined by Beaufort scale and is much lower than the wind speed for normal operation of a large wind farm (~10 m s −1 ), indicating the effectiveness of the TEG in addressing mild agitation from air flow. Second, water flow was successfully demonstrated as a target mechanical source ( Fig. 7b ). The TEG was connected to the central shaft of a miniaturized water turbine (bottom inset in Fig. 7b ). Normal tap water at a flow rate of 5.5 l min −1 was directed into the turbine inlet through a plastic pipe (top inset in Fig. 7b ), which served as a sufficient driving force for the TEG. Consequently, output power for the spot lights was continuously produced ( Supplementary Movie 11 ). Last but not the least, the TEG could also effectively operate if the input mechanical energy originated from gentle body movement. As illustrated in Fig. 7c , the compact-sized TEG in a hand had pieces of inertia mass fixed on the rotator. As the hand swung back and forth in small amplitude, asymmetric inertia resulting from the extra mass induced relative rotation between the hand-held stator and the free-standing rotator. The spot lights again served as an explicit indicator of the produced output power from the TEG ( Supplementary Movie 12 ). 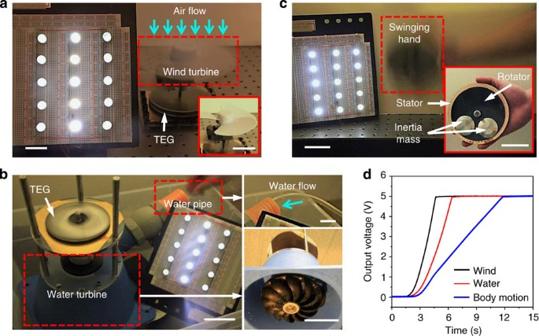Figure 7: Demonstrations of the triboelectric generator for harvesting ambient energy. (a) Harvesting energy from light wind at a flow speed of 6 m s−1by the triboelectric generator for powering an array of spot lights (scale bar, 3 cm). Inset: a wind turbine that transmits torque to the triboelectric generator (scale bar, 5 cm). (b) Harvesting energy from water flow at a flow rate of 5.5 L min−1by the triboelectric generator for powering an array of spot lights (scale bar, 5 cm). Insets: tap water is directed into a water turbine through a water pipe (top; scale bar, 2 cm); upward view of the water turbine (bottom; scale bar, 7 cm). (c) Harvesting energy from body motion by the triboelectric generator that is being gently swung with a hand for powering an array of spot lights (scale bar, 5 cm). Inset: the hand-held triboelectric generator with two pieces of inertia mass attached to the rotator (scale bar, 5 cm). (d) Output voltage of the power-supplying system when the triboelectric generator is driven by the above three types of ambient mechanical energy. Figure 7: Demonstrations of the triboelectric generator for harvesting ambient energy. ( a ) Harvesting energy from light wind at a flow speed of 6 m s −1 by the triboelectric generator for powering an array of spot lights (scale bar, 3 cm). Inset: a wind turbine that transmits torque to the triboelectric generator (scale bar, 5 cm). ( b ) Harvesting energy from water flow at a flow rate of 5.5 L min −1 by the triboelectric generator for powering an array of spot lights (scale bar, 5 cm). Insets: tap water is directed into a water turbine through a water pipe (top; scale bar, 2 cm); upward view of the water turbine (bottom; scale bar, 7 cm). ( c ) Harvesting energy from body motion by the triboelectric generator that is being gently swung with a hand for powering an array of spot lights (scale bar, 5 cm). Inset: the hand-held triboelectric generator with two pieces of inertia mass attached to the rotator (scale bar, 5 cm). ( d ) Output voltage of the power-supplying system when the triboelectric generator is driven by the above three types of ambient mechanical energy. Full size image Furthermore, with input mechanical energy fed from the above ambient motions, the power management circuit was still functional and showed a linearly increasing output voltage as it was being charged up by the TEG ( Fig. 7d ). Therefore, these demonstrations firmly prove that the TEG can fully operate in normal environment by utilizing ambient mechanical energy from a variety of sources, indicating its widespread applications in harvesting human motions and even natural energy. Compared with other existing technologies for power generation, the TEG is distinct in basic mechanism from fundamental point of view. The usual electric generator mostly relies on electromagnetic induction, an effect from the coupling between bulk magnetic materials and conductors. In comparison, our generator depends on triboelectrification, a universally applicable charging effect that is confined only at contact surfaces. Such a distinction in fundamental mechanism differentiates our generator from the traditional generator in a number of major aspects. In general, the TEG is a complementary approach in parallel to the traditional electric generator. Its uniqueness as well as real advantages is elaborated below. From the structure point of view, the usual generator has a bulky structure since the output power heavily depends on such factors as the number of coil turns, the diameter of metal coils, the coil geometry and the size as well as weight of magnets. The shrinkage in size results in substantial deterioration in output power due to insufficient electromagnetic coupling and other parasitic effects [36] . Therefore, the usual generator normally has relatively large size and weight for producing a decent output power. For example, our test on a commercial mini-sized generator of 8.2 cm 3 in volume and 29 g in weight showed an optimum output power of 0.13 W when rotating at 1,800 r min −1 . In comparison, our generator relies on triboelectrification, a surface charging effect. The simple stator–rotator structure has a two-dimensional planar configuration. In addition to using hard sheets as substrates ( Fig. 1 ), we can further extend the substrate materials to plastic thin-film materials that are flexible such as polyimide by using photolithography and laser patterning techniques ( Supplementary Fig. 8 , Methods). Having the same radius and radial periodicity as the device in Fig. 1 , the thin-film TEG gave the same level of output shown in Fig. 2 . It is only 75 μm in total thickness, 0.6 cm 3 in volume, and 1.1 g in weight, similar to the weight of a few goose feathers. From performance point of view, the TEG has substantially higher power density than the traditional generator in terms of both power-to-volume ratio and power-to-weight ratio due to much smaller volume and weight. The high power density imparts two major advantages to practical applications of the TEG. First, it is superior to the conventional generator as a small-sized power source for self-powered electronics, for example, harvesting human motions for powering or charging portable/wearable gadgets. In these applications, size and weight management become critical issues. Second, the significant power density makes the TEG potentially advantageous in large-scale power generation for stationary power plants, although the feasibility needs to be solidly validated with further investigations. From cost point of view, the TEG on the basis of surface charging effect only needs very small amount of materials. They are conventional thin-film insulating materials and metals of various kinds that are abundantly available. Besides, it has a simple structure and straightforward fabrication process. As a consequence, the TEG is extremely cost-effective, which is an unparalleled advantage compared with any other power generation techniques. The significantly low cost of the TEG is a key advantage for its potential widespread applications. Last but not the least, our unique 2-dimensional-planar generator owns distinctive applicability in a variety of circumstances. The usual generator has difficulty being made into a planar structure due to reasons such as poor properties of planar magnets, limited number of turns achievable with planar coils and restricted amplitude of displacement [36] . In comparison, the TEG offers a straightforward and even sole solution to addressing rotation sliding between two surfaces. For example, it can be possibly integrated into a brake system in automotive and other applications where a brake rotor and brake pads have relative contact rotation. Moreover, due to the simple rotator–stator structure, our generator provides a much easier and more convenient way to address common rotating motions. For example, with very little modification, the TEG can take advantage of rotating shafts that are commonly found in transmission systems, as clearly demonstrated in Fig. 7 and corresponding Supplementary Movies 10–12 . Besides, enabled by broad choices of materials, the TEG with particular properties can meet special needs. For instance, it can be fabricated from organic biocompatible materials for healthcare and other bio-related applications. Finally, it is the unique solution when installation space is constrained. Therefore, our generator enables unique applications in many circumstances where the usual generator cannot be implemented, although both of them utilize rotation for power generation. In summary, we developed a new type of planar-structured electricity-generation method (TEG) to convert mechanical energy using triboelectrification effect, a universal phenomenon upon contact between two materials. On the basis of the stator–rotator structure that has arrays of micro-sized radial sectors, the TEG produced significantly high output power for sufficiently powering as well as charging conventional consumer electronics. It could effectively harvest a variety of ambient energy from motions such as air flow, water flow and even body motion. Furthermore, the combination of the TEG and a power management circuit demonstrated the immediate practicability of using the TEG for everyday power needs. Given its exceptional power density, extremely low cost and unique applicability, the TEG presented in this work is a practical approach in converting mechanical motions for self-powered electronics as well as possibly for producing electricity at a large scale. Fabrication of a TEG on hard substrates Stator: (1) Cut a square-shaped acrylic sheet as a substrate with a dimension of 13 cm by 13 cm by 3 mm using a laser cutter; (2) Drill through-holes on edges of the substrate for mounting it on a flat stage by screws; (3) Create trenches on top of the substrate using laser cutting. These trenches define the patterns of the two sets of complementary radial-arrayed electrodes; (4) Deposit a layer of Ti (10 nm) and then a layer of Au (100 nm) on the substrate in sequence using an electron-beam evaporator; (5) Connect two lead wires respectively to the electrodes; (6) Adhere a thin layer of FEP (25 μm) onto the electrode layer. Rotator: (1) Cut a disc-shaped acrylic substrate with through-patterns that consist of radial-arrayed sectors using a laser cutter. The rotator has a diameter of 10 cm and a thickness of 1.5 mm; (2) Drill a through-hole that has a D-profile at the centre of the rotator; (3) Use Ar/O 2 plasma (100 W) to do surface treatment on the substrate for 1 min; (4) Deposit a layer of Ti (10 nm) and then a layer of Cu (200 nm) on the rotator in sequence using a DC sputterer. Experimental setup for electric measurement (1) Mount a rotary motor in an inverted way on a three-dimensional linear positioner; (2) Insert the D-profile shaft of the motor into the central hole of the rotator; (3) Align the rotator and the stator to make them in coaxial alignment by using the linear positioner; (4) Adjust height of the linear positioner so that the rotator and the stator are in contact. Fabrication of a TEG on flexible substrates Stator(1) Cut a disc-shaped polyimide substrate (25 μm) as a substrate using a laser cutter; (2) Use photolithography (negative photoresist) to create exposed windows that define electrodes on the substrate; (3) Deposit metal layer by e-beam evaporation, followed by lift-off process to generate the electrode pattern on the substrate; (4) Connect two lead wires respectively to the electrodes; (5) Adhere a thin layer of FEP (25 μm) on top of the electrode as an electrification layer. Rotator: (1) Cut a disc-shaped polyimide substrate (25 μm) as a substrate with through-patterns that consist of radial-arrayed sectors using a laser cutter; (2) Drill a through-hole that has a D-profile at the centre of the rotator; (3) Use Ar/O 2 plasma (100 W) to do surface treatment on the substrate for 1 min; (4) Deposit a layer of Ti (10 nm) and then a layer of Cu (200 nm) on the rotator in sequence using a DC sputterer. How to cite this article: Zhu, G. et al. Radial-arrayed rotary electrification for high performance triboelectric generator. Nat. Commun. 5:3426 doi: 10.1038/ncomms4426 (2014).